Identification of the functional binding pocket for compounds targeting small-conductance Ca2+-activated potassium channels Small- and intermediate-conductance Ca 2+ -activated potassium channels, activated by Ca 2+ -bound calmodulin, have an important role in regulating membrane excitability. These channels are also linked to clinical abnormalities. A tremendous amount of effort has been devoted to developing small molecule compounds targeting these channels. However, these compounds often suffer from low potency and lack of selectivity, hindering their potential for clinical use. A key contributing factor is the lack of knowledge of the binding site(s) for these compounds. Here we demonstrate by X-ray crystallography that the binding pocket for the compounds of the 1-ethyl-2-benzimidazolinone (1-EBIO) class is located at the calmodulin-channel interface. We show that, based on structure data and molecular docking, mutations of the channel can effectively change the potency of these compounds. Our results provide insight into the molecular nature of the binding pocket and its contribution to the potency and selectivity of the compounds of the 1-EBIO class. Ca 2+ -activated potassium channels, such as small- and intermediate-conductance K + channels (SK and IK), are widely expressed in excitable tissues, including the central nervous system and the cardiovascular system [1] , [2] , [3] , [4] , [5] . They have pivotal roles in regulating membrane excitability by Ca 2+ . Unlike voltage-gated K + channels, activation of SK/IK channels is voltage-independent and is achieved exclusively by Ca 2+ (ref. 6 ). Calmodulin (CaM), constitutively tethered to SK/IK channels, serves as the high-affinity Ca 2+ sensor. Four canonical EF-hands, two located at the CaM N terminus (N-lobe) and the other two at the C terminus (C-lobe), are the high-affinity Ca 2+ -binding domains [7] . Binding of Ca 2+ to CaM results in changes in the CaM conformation and subsequent opening of the channel [8] , [9] , [10] . Both SK and IK channels belong to the same gene family, with four genes identified, KCNN1 for SK1, KCNN2 for SK2, KCNN3 for SK3 and KCNN4 for IK channels [3] , [5] . We have identified an SK2 channel splice variant, SK2-b, which is less sensitive to Ca 2+ for its activation [10] . Activation of SK channels dampens firing of action potentials and therefore contributes to regulation, by Ca 2+ , of neuronal excitability, dendritic integration, synaptic transmission and plasticity in the central nervous system [1] , [3] , [5] , [11] . Equally important are the roles of SK/IK channels in the cardiovascular system [12] , [13] , [14] , [15] . Vascular endothelial cells express both IK and SK3 channels, which contribute to the endothelium-derived hyperpolarizing factor-mediated vasodilation [16] , [17] , [18] , [19] . Increased SK/IK channel activities promote arteriolar vasodilation by enhancing agonist-evoked synthesis of nitric oxide in endothelial cells [20] . The functional importance of SK/IK channels is further demonstrated by their potential involvement in clinical abnormalities [14] , [21] , [22] , [23] . CGA repeats of SK3 channels have been linked to schizophrenia and the bipolar disorder [24] , [25] . Single-nucleotide polymorphisms in the SK/IK genes have been implicated in cardiovascular abnormalities [21] . In the heart, genome-wide association studies reveal a correlation of single-nucleotide polymorphisms of SK3 channels and atrial fibrillation [26] . Compromised SK channel activities may be a contributing factor of hypertension [14] . IK channels are implicated in atherogenesis in mice and human [27] . Recent studies have also suggested the potential link of SK channels and development of cancer, as abnormal expression of SK2 and SK3 channels might contribute to enhanced cell proliferation and cell migration [23] , [28] . Given the roles of SK/IK channels in physiological and pathophysiological conditions, a tremendous amount of effort has been devoted to developing small molecules targeting SK/IK channels [11] , [28] , [29] , [30] , [31] , [32] . 1-EBIO (1-ethyl-2-benzimidazolinone) is such a small molecule prototype, which potentiates the SK/IK channel activities and effectively decreases the neuronal excitability, thus potentially neuroprotective [33] . Indeed, studies on animal models have shown that 1-EBIO can reduce seizure incidence in seizure models [34] and significantly improve survival of hippocampal neurons after cerebral ischaemia [22] . SKA-31, a different channel modulator, enhances the endothelium-derived hyperpolarizing factor-mediated responses and lowers the blood pressure [35] . In general, for compounds of the 1-EBIO class, problems include the low potency and lack of selectivity, which hamper their potential for evaluation in animal models and in clinical trials [2] , [11] . For instance, the half maximal effective concentration (EC50) of 1-EBIO is in the sub-millimolar range for its potentiation of SK2 channels [11] . NS309, although the most potent one of the 1-EBIO class, potentiates both IK and SK channels. CyPPA is relatively more selective, acting on SK2 and SK3 channels, but not on SK1 or IK channels [36] . A key contributing factor is the lack of knowledge of the binding site(s) for these compounds in SK/IK channels, although the channel C terminus is implicated for the action of 1-EBIO [37] . So far, it is not known where or how compounds of the 1-EBIO class interact with SK/IK channels. Here we describe our discovery of the functional binding pocket at the CaM-channel interface of the CaM N-lobe for compounds of the 1-EBIO class, through the combined approaches of X-ray crystallography, molecular docking, mutagenesis and electrophysiology. We also show that phenylurea (PHU) is the most primitive structure of the SK channel modulators of the 1-EBIO class. Our results provide insight into the molecular nature of the binding pocket and its contribution to the potency and selectivity of the compounds of the 1-EBIO class. The knowledge will facilitate development of future generations of therapeutics targeting SK/IK channels. PHU is a weak SK-channel modulator We previously reported that CaM, when complexed with the CaM-binding domain (CaMBD) of a SK2 channel splice variant SK2-b (CaMBD2-b), adopts a drastically different conformation at the CaM C-lobe [10] . Such conformational changes have restored the ability of the CaM C-lobe to bind Ca 2+ ions with reduced affinity, which accounts for the reduced sensitivity of activation of SK2-b channels by Ca 2+ . In solving the structure of the CaM–CaMBD2-b complex (PDB accession code 3SJQ ), it was discovered that PHU, an additive in the crystallization solution, is found at the CaM–CaMBD interface of the CaM N-lobe, but not the CaM C-lobe ( Fig. 1a ). The presence of PHU does not interfere with Ca 2+ -dependent formation of the 2×2 CaM–CaMBD2-b complex [10] . The interaction between PHU and the CaM complex is further confirmed by the protein crystal structure at the resolution of 1.7 Å obtained by soaking in the PHU solution of the CaM–CaMBD2-a complex crystals, which had been grown in the absence of PHU. 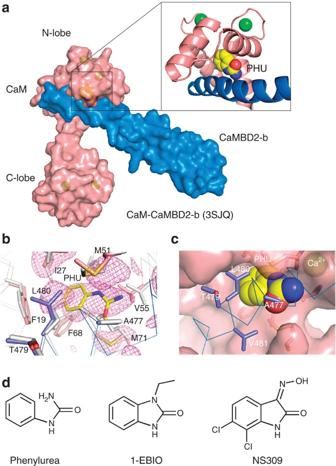Figure 1: Phenylurea (PHU) binds to the CaM–CaMBD interface at the CaM N-lobe. (a) A space-filled model of the CaM–CaMBD2-b complex (3SJQ), depicting the location of PHU (yellow) between the interface of CaM (salmon) and CaMBD2-b (marine) at the CaM N-lobe. Only half of the 2×2 complex is shown for clarity. (b) Difference Fourier electron density map constructed using mFo–DFc coefficients calculated in PHENIX before modelling PHU and side-chain rearrangements that occur in the binding site. The map is contoured at 2.5 σ and displayed within a 6Å sphere of PHU.The map is overlaid with the final coordinates for PHU and its surrounding amino acid residues in the CaM–CaMBD2-a complex. Marine are amino acid residues from CaMBD2-a and salmon are amino acid residues from CaM. Coordinates of the same amino acid residues (grey) from the original CaM–CaMBD2-a complex (without PHU, 1G4Y) are provided for comparison. (c) A space-filled model of PHU at the CaM–CaMBD interface. Marine represents CaMBD and salmon represents CaM. (d) Comparison of the chemical structure of PHU with that of 1-EBIO and NS309. Both 1-EBIO and NS309 are known SK/IK channel modulators. Figure 1: Phenylurea (PHU) binds to the CaM–CaMBD interface at the CaM N-lobe. ( a ) A space-filled model of the CaM–CaMBD2-b complex (3SJQ), depicting the location of PHU (yellow) between the interface of CaM (salmon) and CaMBD2-b (marine) at the CaM N-lobe. Only half of the 2×2 complex is shown for clarity. ( b ) Difference Fourier electron density map constructed using mFo–DFc coefficients calculated in PHENIX before modelling PHU and side-chain rearrangements that occur in the binding site. The map is contoured at 2.5 σ and displayed within a 6Å sphere of PHU.The map is overlaid with the final coordinates for PHU and its surrounding amino acid residues in the CaM–CaMBD2-a complex. Marine are amino acid residues from CaMBD2-a and salmon are amino acid residues from CaM. Coordinates of the same amino acid residues (grey) from the original CaM–CaMBD2-a complex (without PHU, 1G4Y) are provided for comparison. ( c ) A space-filled model of PHU at the CaM–CaMBD interface. Marine represents CaMBD and salmon represents CaM. ( d ) Comparison of the chemical structure of PHU with that of 1-EBIO and NS309. Both 1-EBIO and NS309 are known SK/IK channel modulators. Full size image Structural analysis shows extra electron density, which corresponds to the structure of PHU in the CaM–CaMBD2-a complex ( Fig. 1b ; Supplementary Fig. S1a and b ; Table 1 ). Like the CaM–CaMBD2-b complex ( Fig. 1a ), PHU is located at the interface of CaM–CaMBD2-a of the CaM N-lobe, forming close contacts with both CaM and CaMBD2-a. There are no significant global changes in the structure of the 2×2 configuration of the CaM–CaMBD2-a complex [8] , [10] . The PHU-binding pocket includes A477, L480 and V481 of CaMBD, and F19, I27, L32, M51, I52, V55, I63, F68 and M71 of CaM (within the 5 Å radius of PHU, Fig. 1b,c ; Supplementary Fig. S1 ). Compared with the original structure of CaM–CaMBD2-a (1G4Y) [8] , presence of PHU alters the spatial orientation of amino acids, including L480, F19, M51, V55 and M71 ( Fig. 1b ). Within the binding pocket, the urea group of PHU can adopt two different conformations (flip-flop, Supplementary Fig. S1c ). The most intriguing and unexpected discovery comes from the comparison of the chemical structure of PHU with the known SK/IK channel modulators, such as 1-EBIO and NS309. There is a striking resemblance of the PHU structure to those of 1-EBIO and NS309 ( Fig. 1d ). Table 1 Crystallographic statistics. Full size table To explore whether PHU might act as an SK channel modulator, SK2-a channels were expressed in TsA cells, a transformed human kidney (HEK293) cell line, and their responses to application of PHU were recorded in the presence of 200 nM Ca 2+ in the bath solution [10] . SK2-a channels open upon application of a 200 nM Ca 2+ solution ( Fig. 2a ). The channel activity is further potentiated with increasing PHU concentrations, from 0.2 mM up to 20 mM, with the EC50 of 1.61±0.20 mM and a Hill coefficient of 1.81±0.22 ( n =4). The same experiments were repeated using other known SK channel modulators, such as 1-EBIO, DCEBIO (5,6-dichloro-1-ethyl-1,3-dihydro-2H-benzimidazol-2-one), CyPPA and NS309 (ref. 11 ). Compared with 1-EBIO (EC50=395.5±45.2 μM, n =5), PHU is much less potent in its potentiation of SK2 channels ( P <0.001, Student's t -test, Fig. 2b ). PHU is almost 75-fold less potent than DCEBIO (EC50=21.5±2.7 μM, n =8, Fig. 2c ) and more than 3600-fold less potent compared with NS309 (EC50=0.44±0.13 μM, n =3). CyPPA, which selectively potentiates SK2 and SK3 channels [36] , is ~266-fold more potent than PHU (6.04±1.04 μM, n =6). SK2-b, a SK2 splice variant [10] , and has the same responses as SK2-a to NS309, 0.50±0.09 μM ( n =6, P =0.713, Student's t -test, Fig. 2d ). This demonstrates that SK2-b, although less sensitive to Ca 2+ for its activation [10] , has the same response to the SK channel modulator as SK2-a. 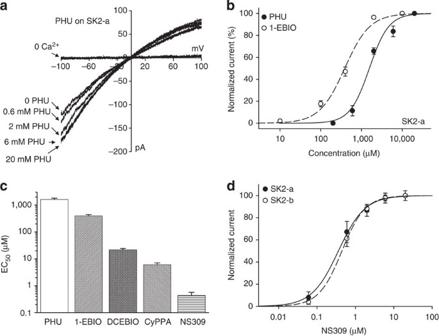Figure 2: Phenylurea (PHU) is a weak SK2 channel modulator. (a) Raw current traces from an inside-out patch with SK2-a channels expressed. The SK2 channels are activated by 200 nM Ca2+, with subsequent potentiation by PHU at the concentrations indicated (all in the presence of 200 nM Ca2+). A voltage ramp, from −100 mV to +100 mV, was applied. (b) Dose–response curves for PHU (n=4) and 1-EBIO (n=5) for their potentiation of the SK2 channel activities (all in the presence of 200 nM Ca2+). The current amplitudes were measured at −90 mV and normalized to the maximal current obtained either with PHU or 1-EBIO. (c) EC50s of potentiation of the SK2 channel activities by PHU (n=4), 1-EBIO (n=5), DCEBIO (n=8), CyPPA (n=6) and NS309 (n=3). All modulators were in a 200 nM Ca2+solution. Note that theyaxis is in the log scale. (d) SK2-a (n=3) and SK2-b (n=6) have the same responses to application of NS309. As SK2-b is less sensitive to Ca2+for its activation, 500 nM Ca2+was used instead of 200 nM Ca2+for SK2-a channels. All data are mean±s.e.m. Figure 2: Phenylurea (PHU) is a weak SK2 channel modulator. ( a ) Raw current traces from an inside-out patch with SK2-a channels expressed. The SK2 channels are activated by 200 nM Ca 2+ , with subsequent potentiation by PHU at the concentrations indicated (all in the presence of 200 nM Ca 2+ ). A voltage ramp, from −100 mV to +100 mV, was applied. ( b ) Dose–response curves for PHU ( n =4) and 1-EBIO ( n =5) for their potentiation of the SK2 channel activities (all in the presence of 200 nM Ca 2+ ). The current amplitudes were measured at −90 mV and normalized to the maximal current obtained either with PHU or 1-EBIO. ( c ) EC50s of potentiation of the SK2 channel activities by PHU ( n =4), 1-EBIO ( n =5), DCEBIO ( n =8), CyPPA ( n =6) and NS309 ( n =3). All modulators were in a 200 nM Ca 2+ solution. Note that the y axis is in the log scale. ( d ) SK2-a ( n =3) and SK2-b ( n =6) have the same responses to application of NS309. As SK2-b is less sensitive to Ca 2+ for its activation, 500 nM Ca 2+ was used instead of 200 nM Ca 2+ for SK2-a channels. All data are mean±s.e.m. Full size image 1-EBIO binds to the same pocket as PHU The above observation led us to test whether, like PHU, SK channel modulators of the 1-EBIO class might also bind to the same CaM–CaMBD interface at the CaM N-lobe. Protein crystals of CaM–CaMBD2-a, grown without SK channel modulators, were soaked in the crystallization solution supplemented with saturating amount of 1-EBIO. The structure of the protein complex with 1-EBIO was resolved at the resolution of 1.7 Å. Again, there exists extra electron density, at the same location of the CaM N-lobe (for example, Fig. 1a ), but not the CaM C-lobe ( Fig. 3a ; Supplementary Fig. S2a ; Table 1 ). Likewise, no significant global changes are observed in the structure of the CaM–CaMBD2-a complex. The 1-EBIO-binding pocket consists of A477, L480 and V481 of CaMBD2-a, and F19, I27, L32, M51, I52, V55, I63, F68, M71 and M72 of CaM (within the 5 Å radius of 1-EBIO), virtually identical to the PHU-binding pocket ( Fig. 3b ). Compared with the structure without 1-EBIO (PDB accession code 1G4Y ), several of these residues display different spatial orientations, most noticeably A477 and L480 of CaMBD and F19, M51, V55 and M71 of CaM ( Fig. 3a ). For instance, in the absence of 1-EBIO or PHU, M71 of CaM forms close contacts with A477 and L480 of CaMBD ( Supplementary Fig. S2b ). Such interactions are completely disrupted by either 1-EBIO or PHU, leading to formation of the binding pocket for 1-EBIO or PHU ( Fig. 3c ; Supplementary Fig. S2c and d ). Depending on whether the ligand is PHU or 1-EBIO, these amino acids may adopt different conformations, for example, L480, F68 and M71, ( Fig. 3b ). Furthermore, the benzene ring of 1-EBIO adopts a different spatial orientation compared with that of PHU ( Fig. 3d ). Unlike PHU, 1-EBIO does not show flip-flop within its binding pocket. 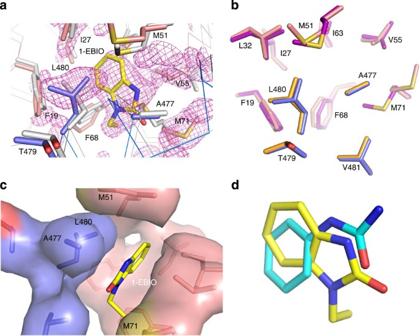Figure 3: The CaM–CaMBD interface harbours the binding pocket for 1-EBIO. (a) Difference Fourier electron density map constructed using mFo–DFc coefficients calculated in PHENIX before modelling 1-EBIO and side-chain rearrangements that occur in the binding site. The map is contoured at 2.2 σ and displayed within a 6 Å sphere of 1-EBIO.The map is overlaid with the final coordinates for 1-EBIO and its surrounding amino acid residues in the CaM–CaMBD2-a complex. Marine are amino acid residues from CaMBD2-a and salmon are amino acid residues from CaM. Coordinates of the same amino acid residues (grey) from the original CaM–CaMBD2-a complex (without 1-EBIO, 1G4Y) are provided for comparison. (b) Comparison of key amino acid residues, which form the binding pocket for PHU (orange for CaMBD residues and purple for CaM residues) and that for 1-EBIO (marine for CaMBD residues and salmon for CaM residues). (c) Formation of the 1-EBIO-binding pocket at the CaM–CaMBD interface. 1-EBIO disrupts the interaction between M71 of CaM (salmon) and A477/L480 of CaMBD (marine). (d) Overlay of the coordinates for 1-EBIO (yellow) and PHU (cyan) obtained from their respective protein crystal structures. Figure 3: The CaM–CaMBD interface harbours the binding pocket for 1-EBIO. ( a ) Difference Fourier electron density map constructed using mFo–DFc coefficients calculated in PHENIX before modelling 1-EBIO and side-chain rearrangements that occur in the binding site. The map is contoured at 2.2 σ and displayed within a 6 Å sphere of 1-EBIO.The map is overlaid with the final coordinates for 1-EBIO and its surrounding amino acid residues in the CaM–CaMBD2-a complex. Marine are amino acid residues from CaMBD2-a and salmon are amino acid residues from CaM. Coordinates of the same amino acid residues (grey) from the original CaM–CaMBD2-a complex (without 1-EBIO, 1G4Y) are provided for comparison. ( b ) Comparison of key amino acid residues, which form the binding pocket for PHU (orange for CaMBD residues and purple for CaM residues) and that for 1-EBIO (marine for CaMBD residues and salmon for CaM residues). ( c ) Formation of the 1-EBIO-binding pocket at the CaM–CaMBD interface. 1-EBIO disrupts the interaction between M71 of CaM (salmon) and A477/L480 of CaMBD (marine). ( d ) Overlay of the coordinates for 1-EBIO (yellow) and PHU (cyan) obtained from their respective protein crystal structures. Full size image Predicted binding pockets for other 1-EBIO compounds Poor solubility of NS309 and CyPPA in water made it difficult to get protein crystals with these compounds. We therefore turned to molecular docking and molecular dynamics (MD) simulations to test whether DCEBIO, NS309 and CyPPA might also fit into the same binding pocket for PHU and 1-EBIO. Both molecular docking and MD simulations were performed using protein coordinates from the PHU-bound CaM–CaMBD structure after removal of PHU. The Generalized-Born with molecular volume (GBMV) implicit solvent model was used to calculate the linear interaction energy (LIE(GBMV)) to score individual poses obtained from docking and MD modelling [38] , [39] . We started by testing whether molecular docking and MD simulations would correctly dock both PHU and 1-EBIO in their respective native conformations determined from the protein crystals ( Figs 1 and 3 ). Both rigid-receptor and 'flexible-receptor' approaches were used to characterize putative binding modes for PHU and 1-EBIO. Rigid-receptor docking is able to successfully re-dock PHU into the PHU pocket with the difference between the experimental and predicted poses of 1.30 Å r.m.s.d. (root-mean square deviation, calculated over 10 heavy atoms). Likewise, 1-EBIO is able to dock into the PHU pocket with low-energy unstrained ligand geometries and favourable LIE(GBMV) scores. The difference of the experimental and predicted poses of 1-EBIO is 2.44 Å r.m.s.d. (calculated over all 12 heavy atoms), which arises primarily from the symmetry-related conformation of the ethyl group of 1-EBIO (5.50 Å r.m.s.d. ), whereas the 10 atoms of the fused ring system only differ by 1.05 ˚Å r.m.s.d. Unlike 1-EBIO, the rigid-receptor docking does not work well in docking both di-chloral compounds (DCEBIO and NS309) into the PHU pocket. The top-ranked binding geometries of these ligands exhibited strained ligand conformations, particularly, the clashes of both ligands with F68, M71 and M72 of CaM, consistent with the observation of the crystal structures that F68 and M71 change their conformation when the ligand is 1-EBIO instead of PHU ( Fig. 3b ). Receptor ensemble docking (RED) was performed using conformations generated from both MD simulations and from low-energy rotamers built from the PHU-bound crystal structure [40] . Top-ranked ligand-pose clusters were identified for each receptor conformation using the LIE(GBMV) scores. Comparison of top-ranked clusters across the ensemble of receptor conformations demonstrated a reasonable consensus ligand-binding geometry for DCEBIO and NS309, such that at least three of the top-five-ranked clusters were within 1.0 Å heavy atom r.m.s.d. from each other. Compared with NS309 and DCEBIO, CyPPA is a much bigger molecule. Nevertheless, rigid-receptor docking works reasonably well and is able to dock CyPPA into the PHU-binding pocket. 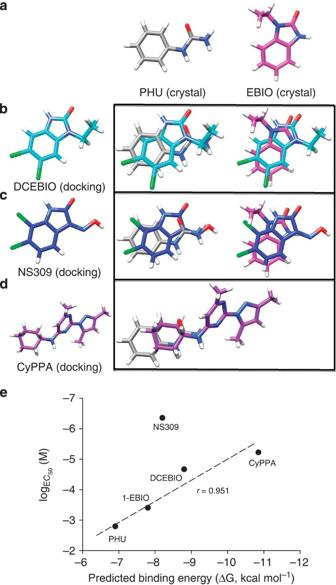Figure 4: Other compounds dock into the same pocket as PHU and 1-EBIO. (a) Conformations of PHU and 1-EBIO determined from the crystal structures. They serve as reference conformations. (b) The predicted conformation of DCEBIO in the binding pocket (left), which is superimposed with the conformations of PHU or 1-EBIO (right). (c) The predicted conformation of NS309 in the binding pocket (left), which is superimposed with the conformations of PHU or 1-EBIO (right). (d) The predicted conformation of CyPPA in the binding pocket (left), which is superimposed with the conformations of PHU or 1-EBIO (right). (e) Correlation of the predicted binding free energies of the five ligands using the S2 scoring function and the EC50s of these compounds in potentiation of SK2 channels. The EC50 for NS309 deviates from the prediction. Figure 4 illustrates the predicted conformations for DCEBIO ( Fig. 4b ), NS309 ( Fig. 4c ) and CyPPA ( Fig. 4d ), and comparison of these conformations to those of PHU and 1-EBIO obtained from crystals ( Fig. 4a ). We also examined whether the NS309 tautomers might have different conformations when docked in the PHU pocket. All three tautomers are predicted to have the same conformation in the PHU pocket ( Supplementary Fig. S3 ). The top-ranked poses of these compounds are further evaluated by a regression-based pair potential (S2-scoring) to predict their binding energy. Qualitatively, there is a positive correlation of the predicted binding energy and the EC50 for each compound in their potentiation of the SK2 channel activities ( Fig. 4e ). Among the five compounds, NS309 is clearly an exception in that it is over 100-fold more potent than the prediction (see Discussion ). Figure 4: Other compounds dock into the same pocket as PHU and 1-EBIO. ( a ) Conformations of PHU and 1-EBIO determined from the crystal structures. They serve as reference conformations. ( b ) The predicted conformation of DCEBIO in the binding pocket (left), which is superimposed with the conformations of PHU or 1-EBIO (right). ( c ) The predicted conformation of NS309 in the binding pocket (left), which is superimposed with the conformations of PHU or 1-EBIO (right). ( d ) The predicted conformation of CyPPA in the binding pocket (left), which is superimposed with the conformations of PHU or 1-EBIO (right). ( e ) Correlation of the predicted binding free energies of the five ligands using the S2 scoring function and the EC50s of these compounds in potentiation of SK2 channels. The EC50 for NS309 deviates from the prediction. Full size image The CaM–CaMBD interface is the functional binding pocket Site-directed mutagenesis was carried out to determine whether the CaM–CaMBD interface at the CaM N-lobe, identified from our structural data ( Figs 1 and 3 ) or predicted by molecular docking ( Fig. 4 ), represents the functional binding pocket for compounds of the 1-EBIO class. Previous studies show that 1-EBIO is more potent in potentiating the IK channel activity than that of SK channels [11] , [33] . In the CaM–CaMBD2-a complex, the channel fragment, E469–Q487, interacts with the CaM N-lobe in the presence of Ca 2+ (refs 8 , 10 ). Sequence alignment of IK and SK shows that of these 19 amino acids, 11 are different between IK and SK2, including A477, L480 and V481, implicated in formation of the binding pocket for PHU or 1-EBIO ( Figs 1 , 3 , 5a ). Mutagenesis studies were performed to test whether mutant channels might respond differently to potentiation by 1-EBIO or other channel modulators. A double mutant, A477V/L480M, was created and its responses to 1-EBIO were tested. A second mutant, T479S, was generated to test whether amino acids, which are different between IK and SK2 but are not involved in formation of the binding pocket for 1-EBIO ( Fig. 3b ), might have any impact on the effects of 1-EBIO. 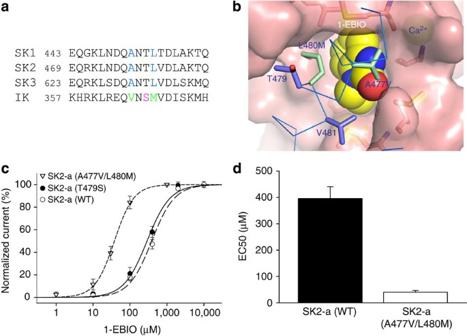Figure 5: A477V/L480M mutation increases the potency of 1-EBIO. (a) Sequence alignment of the fragments (equivalent of E469 to Q487 of SK2-a) of CaMBD at the CaM N-lobe from SK1, SK2, SK3 and IK channels. A477, L480 and V481 are implicated in formation of the binding pocket for the channel modulators from the structure data. Used in the alignment are the human SK1-, SK3- and IK-channel sequences and the rat SK2-channel sequence. (b) A space-filled model of the A477V/L480M mutation (green) with 1-EBIO in the binding pocket. Changes are made based on the structural data using Pymol. Note that T479 points away from 1-EBIO. (c) Dose–response curves for potentiation by 1-EBIO of the SK2 channel activities from WT (n=5), T479S (n=4) and A477V/L480M (n=4); 200 nM Ca2+was present in all 1-EBIO solutions. (d) A477V/L480M mutation significantly increases the potency of 1-EBIO (10-fold,n=4). All data are mean±s.e.m. Figure 5: A477V/L480M mutation increases the potency of 1-EBIO. ( a ) Sequence alignment of the fragments (equivalent of E469 to Q487 of SK2-a) of CaMBD at the CaM N-lobe from SK1, SK2, SK3 and IK channels. A477, L480 and V481 are implicated in formation of the binding pocket for the channel modulators from the structure data. Used in the alignment are the human SK1-, SK3- and IK-channel sequences and the rat SK2-channel sequence. ( b ) A space-filled model of the A477V/L480M mutation (green) with 1-EBIO in the binding pocket. Changes are made based on the structural data using Pymol. Note that T479 points away from 1-EBIO. ( c ) Dose–response curves for potentiation by 1-EBIO of the SK2 channel activities from WT ( n =5), T479S ( n =4) and A477V/L480M ( n =4); 200 nM Ca 2+ was present in all 1-EBIO solutions. ( d ) A477V/L480M mutation significantly increases the potency of 1-EBIO (10-fold, n =4). All data are mean±s.e.m. Full size image Both A477V/L480M and T479S mutants are activated in response to application of 200 nM Ca 2+ . Their responses to application of 1-EBIO, however, differ from each other significantly. The EC50 for potentiation of A477V/L480M by 1-EBIO is 40.0±7.0 μM ( n =4), a 10-fold reduction compared with that of wild-type (WT) SK2-a ( P <0.001, Student's t -test, Fig. 5c,d ). In contrast, the EC50 for potentiation of T479S remains the same as that of WT (EC50=316.8±40 μM, n =4, P =0.245, Student's t -test, Fig. 5c ), consistent with our structure data that T479 is not part of the binding pocket ( Figs 1 , 3 and 5 ). Although A477V/L480M becomes more sensitive to potentiation by 1-EBIO, there is no change in its Ca 2+ -dependent activation (EC50=0.32±0.01 μM, n =3, Supplementary Fig. S4 ). The unique role of A477 was further tested by additional mutants, with the Ala residue replaced by much bulkier amino acid residues, such as Ile or Leu. We reasoned that bulkier residues at position 477 might clash with the channel modulators and therefore interfere with the interaction between the channel modulators and their binding pocket (for example, Fig. 6a,b ). 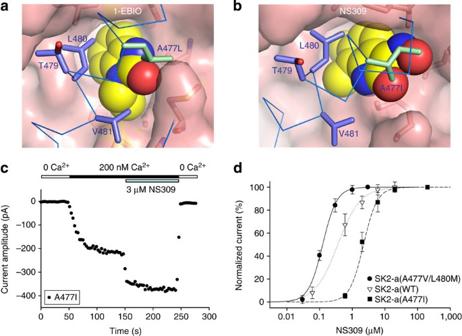Figure 6: Effects of replacing A477 with bulky amino acid residues, Leu and Ile. (a) A space-filled model of the A477L mutation (green) with 1-EBIO in the binding pocket. The Ala residue at position 477 is changed to Leu based on the structural data using Pymol. Introduction of such a bulky amino acid residue may interfere with the interaction of 1-EBIO and its binding pocket. (b) A space-filled model of the A477I mutation (green) with NS309 in the binding pocket. NS309 is docked to the binding pocket using MD modelling from the structure of the 1-EBIO-bound CaM–CaMBD2-a complex. The A477I change is then made using Pymol. (c) Responses of the A477I mutant, from an inside-out patch, to sequential applications of solutions containing (1) 0 Ca2+, (2) 200 nM Ca2+, (3) 3 μM NS309 with 200 nM Ca2+and (4) 0 Ca2+(as indicated). The current amplitudes were measured at −90 mV. (d) Dose–response curves for potentiation by NS309 of the SK2 channel activities from WT (n=3), A477V/L480M (n=4) and A477I (n=3); 200 nM Ca2+was present in all NS309 solutions. On average, the A477V/L480M mutation shifts the NS309 dose–response curve to the left by 3.4-fold, whereas the A477I mutation results in a fivefold shift of the NS309 dose–response curve to the right. All data are mean±s.e.m. Figure 6: Effects of replacing A477 with bulky amino acid residues, Leu and Ile. ( a ) A space-filled model of the A477L mutation (green) with 1-EBIO in the binding pocket. The Ala residue at position 477 is changed to Leu based on the structural data using Pymol. Introduction of such a bulky amino acid residue may interfere with the interaction of 1-EBIO and its binding pocket. ( b ) A space-filled model of the A477I mutation (green) with NS309 in the binding pocket. NS309 is docked to the binding pocket using MD modelling from the structure of the 1-EBIO-bound CaM–CaMBD2-a complex. The A477I change is then made using Pymol. ( c ) Responses of the A477I mutant, from an inside-out patch, to sequential applications of solutions containing (1) 0 Ca 2+ , (2) 200 nM Ca 2+ , (3) 3 μM NS309 with 200 nM Ca 2+ and (4) 0 Ca 2+ (as indicated). The current amplitudes were measured at −90 mV. ( d ) Dose–response curves for potentiation by NS309 of the SK2 channel activities from WT ( n =3), A477V/L480M ( n =4) and A477I ( n =3); 200 nM Ca 2+ was present in all NS309 solutions. On average, the A477V/L480M mutation shifts the NS309 dose–response curve to the left by 3.4-fold, whereas the A477I mutation results in a fivefold shift of the NS309 dose–response curve to the right. All data are mean±s.e.m. Full size image Both A477L and A477I were activated upon application of 200 nM Ca 2+ (for example, Fig. 6c ). A477L was tested for its response to 1-EBIO in the presence of 200 nM Ca 2+ . Even at the saturating concentration of 1-EBIO, we were not able to obtain the maximal response by A477L, indicating that 1-EBIO becomes less potent in potentiation of the A477L mutant (data not shown). We next tested the effects of NS309, a more potent modulator, on these mutants. A477I becomes less responsive to potentiation by NS309 as compared with WT ( Fig. 6c,d ). On average, there is a fivefold increase in the EC50 for A477I (2.21±0.39 μM, n =3), compared with that of WT (0.44±0.13 μM, n =3, P =0.013, Student's t -test). In contrast, when NS309 was tested on A477V/L480M, the EC50 significantly reduced ( Fig. 6d ) to 0.13±0.009 μM ( n =4, P =0.039, Student's t -test, compared with WT). Like A477V/L480M, Ca 2+ -dependent activation of A477I remains the same as WT (EC50=0.33±0.03 μM, n =3). The results suggest that NS309 binds to the same pocket as 1-EBIO, supporting the prediction by molecular docking ( Fig. 4 ). Collectively, mutations, generated based on the structure data, can effectively increase or decrease the potency of both 1-EBIO and NS309, supporting the notion that the binding site, identified by our structure data, is indeed a functional binding pocket for the compounds of the 1-EBIO class. Targeting the CaM-channel interface alters specificity Compared with other compounds of the 1-EBIO class, CyPPA, a much bigger molecule (c.f. Fig. 1d ; Supplementary Fig. S5a ), is more selective, which potentiates SK2 and SK3 channels with little effect on SK1 or IK channels [36] . Molecular docking and MD simulations predicted that CyPPA could bind to the same binding pocket as 1-EBIO ( Figs 4 and 7a ). It was further predicted that the A477V/L480M mutation might change the local environment of the binding pocket and force CyPPA to adopt a different conformation ( Fig. 7b ; Supplementary Fig. S5 ). Such predictions were tested by electrophysiology combined with mutagenesis. CyPPA is reasonably potent (EC50=6.04±1.04 μM, n =6, Fig. 2c ). However, the response of A477V/L480M to CyPPA is distinctively different from that of 1-EBIO ( Fig. 5c ). A477V/L480M barely increases its current amplitude upon application of 100 μM CyPPA ( Fig. 7c,d ). Subsequent application of NS309 produces robust potentiation ( Fig. 7c ), indicating that A477V/L480M has virtually lost its response to CyPPA. In contrast, V481T yields an EC50 of 5.29±1.01 μM ( n =3) for CyPPA, same as the WT ( P =0.666, Student's t -test). The results again support the prediction, by molecular docking, that the binding site at the CaM–CaMBD interface, identified by our structure data, is the functional binding pocket for compounds of the 1-EBIO class. Furthermore, mutations A477V/L480M mimicks the selective effect of CyPPA on IK channels. 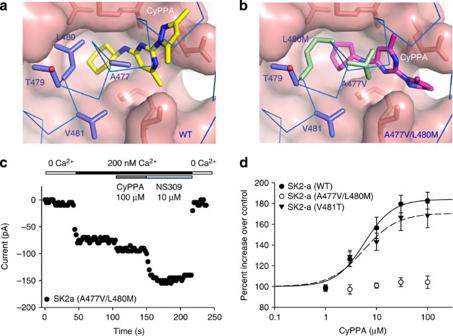Figure 7: Responses of the A477V/L480M mutation to application of CyPPA. (a) A space-filled model of CyPPA docked into the binding pocket. Molecular docking and MD simulation were performed to dock CyPPA into the PHU-binding pocket based on the structure of PHU in the CaM–CaMBD2-a complex. (b) A space-filled model of CyPPA docked into the binding pocket with the A477V/L480M mutation (green). Molecular docking and MD simulations were performed to introduce the A477V/L480M mutation and then docking of CyPPA. Note that the A477V/L480M mutation is predicted to force CyPPA to adopt a different conformation in the pocket. (c) The A477V/L480M mutation on the effect of CyPPA. Responses of the A477V/L480M mutant, from an inside-out patch, to sequential application of solutions containing (1) 0 Ca2+, (2) 200 nM Ca2+, (3) 100 μM CyPPA with 200 nM Ca2+, (4) 10 μM NS309 with 200 nM Ca2+and (5) 0 Ca2+. The current amplitudes were measured at −90 mV. Note that CyPPA, at 100 μM, barely potentiates the mutant channel activity. (d) Responses of SK2 channels, WT (n=6), V418T (n=3) and A477V/L480M (n=5), to increasing concentrations of CyPPA; 200 nM Ca2+was present in all CyPPA solutions. Note that there is little response from the A477V/L480M mutant at the CyPPA concentration range tested. All data are mean±s.e.m. Figure 7: Responses of the A477V/L480M mutation to application of CyPPA. ( a ) A space-filled model of CyPPA docked into the binding pocket. Molecular docking and MD simulation were performed to dock CyPPA into the PHU-binding pocket based on the structure of PHU in the CaM–CaMBD2-a complex. ( b ) A space-filled model of CyPPA docked into the binding pocket with the A477V/L480M mutation (green). Molecular docking and MD simulations were performed to introduce the A477V/L480M mutation and then docking of CyPPA. Note that the A477V/L480M mutation is predicted to force CyPPA to adopt a different conformation in the pocket. ( c ) The A477V/L480M mutation on the effect of CyPPA. Responses of the A477V/L480M mutant, from an inside-out patch, to sequential application of solutions containing (1) 0 Ca 2+ , (2) 200 nM Ca 2+ , (3) 100 μM CyPPA with 200 nM Ca 2+ , (4) 10 μM NS309 with 200 nM Ca 2+ and (5) 0 Ca 2+ . The current amplitudes were measured at −90 mV. Note that CyPPA, at 100 μM, barely potentiates the mutant channel activity. ( d ) Responses of SK2 channels, WT ( n =6), V418T ( n =3) and A477V/L480M ( n =5), to increasing concentrations of CyPPA; 200 nM Ca 2+ was present in all CyPPA solutions. Note that there is little response from the A477V/L480M mutant at the CyPPA concentration range tested. All data are mean±s.e.m. Full size image This study represents the first to demonstrate the location of the functional binding pocket for compounds of the 1-EBIO class. Several lines of evidence support this conclusion. First, PHU, a weak SK2 channel modulator, is found in the identical location at the CaM–CaMBD interface obtained from two CaMBD splice variants, CaMBD2-b and CaMBD2-a, under two different conditions to grow the protein crystals: co-crystallization or soaking of the naive crystals in the PHU solution. Second, 1-EBIO is found to be at the same location as PHU in the CaM–CaMBD complex. Third, both PHU and 1-EBIO pockets are found at the CaM N-lobe, but not at the CaM C-lobe, despite the same hydrophobic nature of the CaM–CaMBD interface at the CaM C-lobe, indicating the specificity of the interaction between PHU/1-EBIO and their binding pockets. Fourth, mutations of amino acids, which form the binding pocket, can change the potency of 1-EBIO, NS309 and CyPPA. Finally, mutations of amino acids not involved in formation of the binding pocket have the same responses to 1-EBIO or CyPPA as WT. The results are also consistent with a previous report that the channel C terminus is responsible for the action of 1-EBIO [37] . With few exceptions, compounds of the 1-EBIO class have low potency, with EC50s up to hundreds of micromolars in their potentiation of SK channels (see ref. 11 for a list of EC50s by different compounds). The low potency also contributes to the poor therapeutic index for these compounds [2] , [34] . Thus far, NS309 is the most potent SK/IK channel modulator, with the EC50 in the sub-micromolar range ( Fig. 2c ). Clearly, chemical modification of the compound has led to such a dramatic improvement in the potency [41] . Identification of the functional binding pocket allows us to evaluate whether the environment of the binding pocket may also have a role in determining the potency of compounds of the 1-EBIO class. Indeed, mutations, such as A477V/L480M and A477I, can significantly alter the potency of 1-EBIO or NS309 (for example, Figs 5 and 6 ). Molecular docking allows us to put DCEBIO, NS309 and CyPPA in the same binding pocket ( Fig. 4 ), and the results of molecular docking are corroborated by effects of mutations on the effectiveness of NS309 and CyPPA ( Figs 6 and 7 ). Molecular docking and MD modelling further show, qualitatively, a correlation of improved interactions of the compounds with the binding pocket and their potency for PHU, 1-EBIO, DCEBIO and CyPPA ( Fig. 4 ). NS309, however, is an exception, with its potency over 100-fold higher than the prediction ( Fig. 4 ). NS309 is likely to bind to the same binding pocket as 1-EBIO, as both A477V/L480M and A477I mutants change the potency of NS309 ( Fig. 6 ). Molecular docking puts NS309 in a somewhat different position from that of 1-EBIO ( Fig. 4c ). Three potential scenarios may explain why NS309 is an outlier in Fig. 4e . First, the NS309 binding pocket may include some additional amino acids from CaMBD and/or CaM, which do not contribute to formation of the PHU pocket or the 1-EBIO pocket used for molecular docking and MD simulations. Second, interactions of NS309 with its binding pocket may stabilize the CaM–CaMBD complex, as demonstrated by a recent study [9] . Such stabilizing effects are not reflected in our estimation of the binding energy (ΔG, Fig. 4e ), which describes only the direct interaction between NS309 and the protein complex. Finally, it is also likely that different NS309 tautomers may have different effects on potentiation of the SK/IK channel activities, although this is a less likely scenario, as molecular docking shows that all three tautomers have the same conformation ( Supplementary Fig. S3 ). Collectively, our results demonstrate that understanding of how compounds, such as 1-EBIO and NS309, interact with the binding pocket will shed light on how to improve the potency of the compounds of the 1-EBIO class. Selectivity is another issue, which hinders the development of more effective therapeutics targeting SK/IK channels [11] , [28] , [29] , [30] , [31] , [32] . With the exception of CyPPA, compounds of the 1-EBIO class as well as toxins, such as apamin, generally lack selectivity amongst SK1, SK2, SK3 and IK channels [36] . Lack of the knowledge of how compounds of the 1-EBIO class interact with their binding sites is likely to be a major roadblock to successful development of more selective therapeutics. The A477V/L480M mutation not only enhances the potency of 1-EBIO by 10-fold ( Fig. 5 ), but also becomes almost insensitive to potentiation by CyPPA ( Fig. 7 ), mimicking the profile of CyPPA on IK channels [36] . However, the results of the A477V/L480M mutation do not explain why SK1 channels fail to respond to CyPPA. Nevertheless, our results show the binding pocket, identified by our protein crystal structures, is at least partially responsible for the selectivity of CyPPA. Protein–protein interactions and formation of macromolecular protein complexes are primary means of efficiency and specificity in cellular signalling [42] . Development of small molecular weight therapeutics targeting the interface of protein–protein interactions represents a new direction of drug discovery, with the biggest advantage of achieving selective actions on targets, which are otherwise too common or widely distributed in cellular signalling [43] , [44] , [45] , [46] . Typically, the protein–protein interface is fairly large (~700–4,000 Å 2 ), and the size differences make it impossible for small molecules to completely block the protein–protein interactions, such as the traditional agonists/antagonists. Within the protein–protein interface, smaller regions, or 'hotspots', are responsible for a disproportionate contribution to the binding energy of the two interacting proteins and are targets for therapeutics [44] , [45] . Our structural data show that the binding pocket for PHU and 1-EBIO includes L480 ( Figs 1 and 3 ), which is the anchor residue interacting with the CaM hydrophobic pocket [8] , [10] , an important hotspot for the CaM–CaMBD interaction [47] , [48] . Thus, compounds of the 1-EBIO class represent another example targeting the protein–protein interface with biological consequences. Understanding the nature of how 1-EBIO and its related compounds interact with the binding pocket will help develop compounds with better potency and selectivity, targeting not only SK/IK channels but also other CaM-target protein complexes involved in Ca 2+ -dependent signalling [47] , [49] , [50] , [51] . Protein expression and purification Briefly, rat CaM cDNA was cloned into pET-28b (Novagen), expressed in E. coli strain Rosetta2(DE3) (Novagen). CaM was purified using a low substitution phenyl sepharose fast-flow column and an AKTA purifier (GE Healthcare). The codons of the CaMBD2-a were optimized for expression in E. coli and the synthetic gene was cloned into pET-28b. The sequence of CaMBD2-a used for expression is: MGRKLELTKAEKHVHNFMMDTQLTKRVKNAAANVLRETWLIYKNTKLVKKIDHAKVRKHQRKF LQAIHQLRSVKMEQRKLNDQANTLVDLAKTQLEHHHHHH. The His-tagged CaMBD2-a was expressed, solubilized with 0.2% w/v sarkosyl and purified on a nickel column (Qiagen). Both CaM and CaMBD2-a were subsequently purified a using Sephacryl S-100 high-resolution gel filtration column (GE Healthcare). The protein concentrations were determined using predicted extinction coefficients. The CaM–CaMBD2-a protein complex was formed by slowly adding the CaMBD2-a to CaM (at a final ratio of 1/1). The complex was then purified using the gel-filtration column (GE Healthcare) pre-equilibrated in a solution with 10 mM Tris–HCl, 150 mM NaCl and 10 mM CaCl 2 (pH 7.5). Fractions were collected and the purified proteins were concentrated to 1 mM and stored at −80 °C. Crystallization and structure determination Protein crystals of the CaM–CaMBD2-a complex were grown in hanging drops by vapour diffusion at 20 °C [8] , [10] . The complex (1 mM) was mixed in a 1/1 ratio with the reservoir solution, which consists of 1.25 M Li 2 SO 4 , 0.5 M (NH 4 ) 2 SO 4 , 0.1 M sodium citrate, pH 5.6. Monoclinic crystals grew within 3 weeks. These preformed protein crystals were then incubated with SK channel modulators at their saturating concentrations for 2 days. The channel modulator-soaked protein crystals were flash-cooled in liquid nitrogen for data collection, after a brief transfer to a suitable cryoprotectant (reservoir solution saturated with SK channel modulators, supplemented by 25% glycerol). X-ray diffraction data were collected from single protein crystals at Beamline of the National Synchrotron Light Source (Brookhaven National Laboratory, Upton, NY, USA) and at the SYBILS Beamline 12.3.1 at the Advanced Light Source (Berkeley, CA, USA) and were processed using Xia2 (ref. 52 ). The CaM–CAMBD2-a complex structure determined in the absence of SK channel agonists (1G4Y) [8] was used as a starting model to phase diffraction data. Solvent molecules were removed from the starting molecule before rigid body refinement against the channel modulator-soaked diffraction data. The crystallographic model was further constructed through iterative rounds of manual model-building using Coot [53] and crystallographic refinement using REFMAC5 [54] and PHENIX [55] . The SK channel modulators were modelled in a hydrophobic pocket of the N-lobe of CaM, based on strong electron density in different Fourier maps, and successful refinement of the coordinates. The current refined models contain CaM residues 2 to 147 with two Ca 2+ ions, and contain SK channel residues 395 to 404 and 413 to 489. Crystallographic statistics for data collection and model refinement are summarized in Table 1 for both models. Structure graphics were created using PyMol (Schrödinger, LLC). Molecular docking CHARMM-based molecular docking is performed for an all-atom force field potential energy description of the protein–ligand complexes [56] , [57] , [58] . The GBMV implicit solvent model was used in the calculation of 'LIE(GBMV)' scores to ensure physically rigorous evaluation of electrostatic potential energy components for the evaluation of top-ranked ligand poses as described previously [38] , [39] . A two-step scoring approach for CHARMM-based molecular docking was used, where the LIE(GBMV) scoring function was used for the identification of the top-ranked ligand-pose geometry, and then a regression-based pair potential (S2) was used to predict binding affinities for ranking compounds [59] . Both rigid-receptor and 'flexible-receptor' approaches were used to characterize putative binding modes for five ligands, PHU, 1-EBIO, DCEBIO, NS309 and CyPPA. Flexible-receptor docking models were initially developed from the structure of PHU-bound CaM–CaMBD, and later compared with the 1-EBIO-bound structure. Short 100-ps MD simulations were performed from the structure of PHU-bound CaM–CaMBD using the GBMV implicit solvent model [38] . Similar MD simulations were also performed from some top-ranked predicted binding modes of 1-EBIO, DCEBIO and NS309, to generate an ensemble of flexible receptor models. For the ensemble of flexible receptors derived from the PHU-bound structure and from MD simulations, 15 total conformations were used, each of which is generated from the final minimized structure from short 100-ps MD simulations of top-ranked binding posed of DCEBIO (5 conformations) and NS309 (10 conformations). An ensemble of rigid-receptor models was also constructed from the PHU-bound crystal structure using the most energetically favourable rotamers of M71 and M72, and F68 (backbone-dependent DUNBRACK library) [60] . The rigid-receptor ensemble constructed from rotamers had 29 members, containing 9 rotamers of M71, 11 rotamers of M72 and 6 rotamers of F68, and finally, three low-energy conformations formed from low-energy-optimized combinations of M71 and M72. RED was then performed assuming that each individual conformation was a rigid receptor [40] . RED was performed using the ensemble of flexible-receptor conformations generated from MD (15 conformations) and low-energy side-chain rotamers built from the crystal structure (29 conformations). Molecular docking was also used to characterize the effect of binding of the ligands to mutations modelled from the PHU-bound structure using all energetically favourable rotamers (backbone-dependent DUNBRACK library) [60] . Mutations, such as A477M/L480M, A477L and A477I, were also modelled using the PHU-bound crystal structure as previously described [60] . Electrophysiology Details can be found in our previous papers [10] . Briefly, both SK2-a and SK2-b channels (WT), along with CaM, were subcloned into the pCDNA3.1 expression vector (Invitrogen), respectively. Mutations were introduced into SK2-a using the QuickChange XL site-directed mutagenesis kit (Stratagene-Agilent) and subsequently confirmed by DNA sequencing. All SK channel modulators were from Tocris, except CyPPA, which was from Sigma-Aldrich. WT and mutant channels, along with CaM and green fluorescent protein, were expressed in TsA201 cells cultured in the DMEM, with 10% fetal bovine serum, and penicillin and streptomycin. A calcium–phosphate method was used for transfection of SK2 cDNA (WT or mutants), together with CaM and green fluorescent protein at a ratio of 5/2.5/1 (weight). Channel activities were recorded 1–2 days after transfection, with a Multiclamp 700B or an Axon200B amplifier (Molecular Devices) at room temperature. pClamp 10.2 (Molecular Devices) was used for data acquisition and analysis. The resistance of the patch electrodes ranged from 3–7 MΩ. The pipette solution contained 140 mM KCl, 10 mM HEPES, 1 mM MgSO 4 , at pH 7.4. The bath solution contained 140 mM KCl and 10 mM HEPES, at pH 7.2. EGTA (1 mM) and HEDTA (1 mM) were mixed with Ca 2+ to obtain 0.2 μM free Ca 2+ , calculated using the software by Chris Patton of Stanford University ( http://www.stanford.edu/~cpatton/maxc.html ). The Ca 2+ concentrations were verified using Fluo-4 and standard Ca2+ buffers (Molecular Probes). Currents were recorded using an inside-out patch configuration. For SK2-a and its mutants, the intracellular face was initially exposed to a zero-Ca 2+ bath solution, and subsequently to bath solutions with 0.2 μM Ca 2+ . Currents were recorded by repetitive 1-s-voltage ramps from −100 mV to +100 mV from a holding potential of 0 mV. One minute after switching of bath solutions, ten sweeps with a 1-s interval were recorded at concentrations for the channel modulators in the presence of 0.2 μM Ca 2+ . For SK2-b channel, a 0.5 μM Ca 2+ solution was used instead of 0.2 μM, because of its reduced Ca 2+ sensitivity for channel activation [10] . The integrity of the patch was examined by switching the bath solution back to the zero-Ca 2+ buffer. Data from patches, which did not show significant changes in the seal resistance after solution changes, were used for further analysis. To construct the dose-dependent potentiation of channel activities, the current amplitudes at −90 mV in response to various concentrations of a channel modulator were normalized to that obtained at maximal concentration. The normalized currents were plotted as a function of the concentrations of each channel modulator. EC50s and Hill coefficients were determined by fitting the data points to a standard dose–response curve ( Y =100/(1+(X/EC50)^−Hill)). Statistical analysis All data are presented in mean±s.e.m. The Student's t -test is used for data comparison. Acccession codes: The atomic coordinates have been deposited in the Protein Data Bank under accession codes 3SJQ , 4G27 and 4G28 for the CaM–CaMBD2-b complex, PHU-bound CaM–CaMBD2-a complex and the 1-EBIO-bound CaM–CaMBD2-a complex, respectively. How to cite this article: Zhang, M. et al . Identification of the functional binding pocket for compounds targeting small-conductance Ca 2+ -activated potassium channels. Nat. Commun. 3:1021 doi: 10.1038/ncomms2017 (2012).